Phosphorylation of BLUS1 kinase by phototropins is a primary step in stomatal opening Opening of stomata in the plant facilitates photosynthetic CO 2 fixation and transpiration. Blue-light perception by phototropins (phot1, phot2) activates the plasma membrane H + -ATPase, causing stomata to open. Here we describe a regulator that connects these components, a Ser/Thr protein kinase, BLUS1 ( BLU E LIGHT S IGNALING 1 ), which mediates a primary step for phototropin signalling in guard cells. blus1 mutants identified by infrared thermography result in a loss of blue light-dependent stomatal opening. BLUS1 encodes a protein kinase that is directly phosphorylated by phot1 in vitro and in vivo at Ser-348 within its C-terminus. Both phosphorylation of Ser-348 and BLUS1 kinase activity are essential for activation of the H + -ATPase. blus1 mutants show lower stomatal conductance and CO 2 assimilation than wild-type plants under decreased ambient CO 2 . Together, our analyses demonstrate that BLUS1 functions as a phototropin substrate and primary regulator of stomatal control to enhance photosynthetic CO 2 assimilation under natural light conditions. Sophisticated control mechanisms optimize stomatal aperture and allow land plants to occupy habitats in ever changing environments [1] , [2] . Stomatal aperture is regulated by light, water status, the phytohormone abscisic acid, CO 2 and other environmental factors, and optimizes plant growth at a given location [3] , [4] , [5] , [6] . Opening of stomata, which is efficiently induced by blue light (BL; 390–500 nm), is achieved by the swelling of guard cells that form the stomatal pore [6] . These specialized cells, in which all biological events required for stomatal opening, including light perception, H + -ATPase activation, K + uptake and swelling of guard cells, occur in a single cell, offer an excellent model system to investigate how light drives reversible cell expansion through changes in solute transport across the membranes. BL is perceived by phototropins (phot1 and phot2), which comprise a small family of light-activated protein kinases associated with the plasma membrane [7] , [8] . Phototropins contain two photoreceptive domains called LOV1 (light, oxygen or voltage) and LOV2 close to the N-terminus, and a C-terminal Ser/Thr kinase. Illumination of plant cells with BL results in phototropin autophosphorylation, an event that is prerequisite for phototropin-mediated responses such as phototropism, chloroplast movements, leaf flattening and stomatal opening [8] , [9] , [10] . However, the mechanisms by which phototropin transduces the light signal into downstream responses are largely unknown. In guard cells, the driving force for stomatal opening is generated by plasma membrane H + -ATPases that are activated via phototropins [11] , [12] , [13] , and it has been established that protein phosphatase 1 (PP1) mediates the signalling between these two molecules [14] . However, the initial signalling event that couples photoreception to activation of the H + -ATPase has yet to be clarified. Genetic dissection of the components involved in this pathway has proven challenging as no reliable method exists to screen for mutants in BL-specific responses in guard cells. We therefore developed a screening strategy to isolate Arabidopsis mutants defective in BL-dependent stomatal opening. Using this tool, we obtained mutants and demonstrate that a novel Ser/Thr protein kinase undergoes phosphorylation as an initial step of phototropin signalling. blus1 mutants lose stomatal responses to BL Using an infrared thermograph [15] , [16] , we constructed a device to monitor changes in leaf temperature in response to BL, and observed the expected temperature decreases resulting from transpiration. Application of weak BL (5 μmol m −2 s −1 ), superimposed on a background of red light (RL; 80 μmol m −2 s −1 ), decreased leaf temperature by 0.6 °C in wild-type (WT) plants but not in the phot1 phot2 double mutant ( Fig. 1a ). This temperature decrease paralleled an increase in stomatal conductance triggered by BL ( Fig. 1b ). Consistent with the different photosensitivities reported previously [11] , phot1 and phot2 single mutants exhibited temperature decreases with low and high sensitivity to BL, respectively ( Supplementary Fig. S1 ). This confirmed that the thermal imaging approach is valid for identifying mutants defective in BL-dependent stomatal opening. 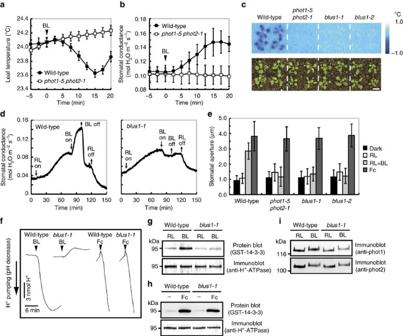Figure 1: Mutations inBLUS1impair stomatal responses to BL. (a,b) Changes of leaf temperature (a) and stomatal conductance (b) in response to BL. Leaves were illuminated by RL (80 μmol m−2s−1) for 50 min, and weak BL (5 μmol m−2s−1) was superimposed. Bars represent means±s.e.m. (n=5). (c) Thermal images of Arabidopsis leaves from WT plants,phot1 phot2andblus1mutants responding to BL. Images were obtained by subtracting an image taken before BL from one taken 15 min after BL. Lower panels show the plants. The bar represents 1 cm. (d) Light-dependent changes in stomatal conductance of intact leaves from wild-type andblus1mutant. RL (600 μmol m−2s−1) and BL (5 μmol m−2s−1) were turned on and off as indicated. (e) Light- and Fc-dependent stomatal opening in the epidermis from WT and mutant plants. Epidermal strips from dark-adapted plants were illuminated with RL (50 μmol m−2s−1) with or without BL (10 μmol m−2s−1) for 2 h. Fc was added to the epidermis at 10 μM. Bars represent means±s.d. (n=75, pooled from triplicate experiments). (f) BL- and Fc-dependent H+pumping in guard cell protoplasts from WT plants andblus1mutants. Guard cell protoplasts were illuminated by RL (600 μmol m−2s−1) for 2 h, and a pulse of BL (100 μmol m−2s−1, 30 s) was applied as indicated. Ten micromolar Fc was used. (g,h) BL- (g) and Fc-dependent (h) phosphorylation of the H+-ATPase in guard cell protoplasts. Phosphorylation of the H+-ATPase was determined by protein blotting using a 14-3-3 protein. Each lane contained 1.5 and 3.5 μg of guard cell proteins for protein blotting (upper panels) and immunoblotting (lower panels). (i) BL-dependent phosphorylation of phototropins (phot1, phot2). The autophosphorylation of phototropins was determined by the upward electrophoretic mobility shift using anti-phot1 and anti-phot2 antibodies. Each lane contained 5 μg of guard cell proteins. Figure 1: Mutations in BLUS1 impair stomatal responses to BL. ( a , b ) Changes of leaf temperature ( a ) and stomatal conductance ( b ) in response to BL. Leaves were illuminated by RL (80 μmol m −2 s −1 ) for 50 min, and weak BL (5 μmol m −2 s −1 ) was superimposed. Bars represent means±s.e.m. ( n =5). ( c ) Thermal images of Arabidopsis leaves from WT plants, phot1 phot2 and blus1 mutants responding to BL. Images were obtained by subtracting an image taken before BL from one taken 15 min after BL. Lower panels show the plants. The bar represents 1 cm. ( d ) Light-dependent changes in stomatal conductance of intact leaves from wild-type and blus1 mutant. RL (600 μmol m −2 s −1 ) and BL (5 μmol m −2 s −1 ) were turned on and off as indicated. ( e ) Light- and Fc-dependent stomatal opening in the epidermis from WT and mutant plants. Epidermal strips from dark-adapted plants were illuminated with RL (50 μmol m −2 s −1 ) with or without BL (10 μmol m −2 s −1 ) for 2 h. Fc was added to the epidermis at 10 μM. Bars represent means±s.d. ( n =75, pooled from triplicate experiments). ( f ) BL- and Fc-dependent H + pumping in guard cell protoplasts from WT plants and blus1 mutants. Guard cell protoplasts were illuminated by RL (600 μmol m −2 s −1 ) for 2 h, and a pulse of BL (100 μmol m −2 s −1 , 30 s) was applied as indicated. Ten micromolar Fc was used. ( g , h ) BL- ( g ) and Fc-dependent ( h ) phosphorylation of the H + -ATPase in guard cell protoplasts. Phosphorylation of the H + -ATPase was determined by protein blotting using a 14-3-3 protein. Each lane contained 1.5 and 3.5 μg of guard cell proteins for protein blotting (upper panels) and immunoblotting (lower panels). ( i ) BL-dependent phosphorylation of phototropins (phot1, phot2). The autophosphorylation of phototropins was determined by the upward electrophoretic mobility shift using anti-phot1 and anti-phot2 antibodies. Each lane contained 5 μg of guard cell proteins. Full size image We screened ethyl methanesulfonate-mutagenized lines and identified two allelic mutants. We named them as blus1-1 and -1-2 ( blu e light s ignaling 1 ), because they shared characteristic phenotypes with a BL-induced slight increase of leaf temperature ( Fig. 1c ). Stomatal conductance in intact leaves gradually increased under strong RL (600 μmol m −2 s −1 ) and reached a steady state. Upon BL illumination (5 μmol m −2 s −1 ), stomatal conductance increased rapidly in the WT and decreased when the illumination had ended ( Fig. 1d ); the blus1 mutants failed to exhibit this blue-light response. Stomata in the epidermis of blus1 mutants were unresponsive to BL, but opened after the application of fusicoccin (Fc), an activator of the H + -ATPase ( Fig. 1e ). Guard cell protoplasts from WT plants showed H + -pumping activity, demonstrated by the acidification of the medium in response to BL [17] . In contrast, blus1 mutant protoplasts slightly alkalized the medium under BL. Yet, similar acidification rates were induced in WT and blus1 plants by Fc ( Fig. 1f ). Intriguingly, the plasma membrane H + -ATPase was phosphorylated in WT but not blus1 plants in response to BL ( Fig. 1g ), whereas similar H + -ATPase phosphorylation was found in WT and blus1 following Fc treatment ( Fig. 1h ). The activities of phot1 and phot2, as determined by a phosphorylation-dependent mobility shift assay, were not impaired in guard cells of blus1 ( Fig. 1i ). On the basis of these results, we concluded that blus1 mutants were specifically defective in the signalling pathway between phototropins and plasma membrane H + -ATPases. It is also noteworthy that blus1 mutants differ phenotypically from phot1 phot2 double mutant. blus1 mutants responded to BL by slight stomatal closure ( Fig. 1c ) and medium alkalization by guard cell protoplasts ( Fig. 1f ). These responses were absent in phot1 phot2 (refs 18 , 19 ), suggesting that a separate phototropin pathway that is independent of BLUS1 is present in guard cells, and may delay stomatal opening through some feedback mechanism. BLUS1 encodes a novel protein kinase Except for stomatal opening, blus1 mutants were not impaired in phototropin-mediated responses, including phototropism, chloroplast movements and leaf flattening ( Supplementary Fig. S2 ). Mutations in the BLUS1 gene were identified by map-based cloning and mapped to the central part of chromosome 4 ( Fig. 2a ). Sequencing of this region in blus1-1 and - 1-2 mutants revealed that At4g14480, which encodes a novel Ser/Thr protein kinase, had point mutations at nucleotides 580 and 574, resulting in substitutions of Lys for Glu-194 and Thr for Ala-192, respectively ( Fig. 2b ). BLUS1 comprises 487 amino acids with a deduced molecular mass of 54.4 kDa, harbouring the E194K for blus1-1 and A192T for blus1-2 mutations within the kinase activation loop in the N-terminus. We generated antibodies against the BLUS1 protein using the C-terminal region of BLUS1. Immunological analysis indicated that the missense mutation lines of blus1-1 and - 1-2 produced BLUS1 proteins that had lost signalling function, and that the T-DNA insertion lines of blus1-3 and blus1-4 were null mutants ( Fig. 2c ). Accordingly, these two mutants were defective in leaf temperature decreases and stomatal opening in response to BL ( Fig. 2d ). A GFP-BLUS1 transgene complemented the blus1-1 mutant phenotype and restored BL-dependent decreases in leaf temperature ( Fig. 2f ). The subcellular localization of GFP:BLUS1 was investigated using complemented lines, in which GFP-BLUS1 was localized to the cytosol ( Fig. 2g ). Furthermore, RT–PCR analyses revealed that BLUS1 was expressed in guard but not mesophyll cells ( Fig. 2h ), which corroborates previous microarray data [20] . 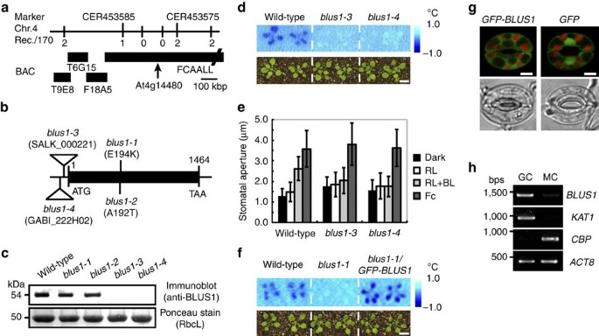Figure 2: Identification of theBLUS1gene. (a) Map-based cloning of theBLUS1gene.BLUS1was mapped to the 290 kbp region between markers CER453585 and CER433575 on BAC clone FCAALL. Numbers indicate the recombination from a total of 170 chromosomes. (b) Genomic structure of theBLUS1gene and sites ofblus1mutations. Black box indicates the protein-coding region. (c) Immunoblot analysis of BLUS1 protein in theblus1mutants. The Rubisco large subunit (RbcL) was used as the loading control. Each lane contained 5 μg of guard cell proteins. (d) Impairment of the BL-dependent leaf temperature decrease of theblus1T-DNA insertion mutants. The bar represents 1 cm. (e) Impairment of the BL-dependent stomatal opening in the epidermis of the T-DNA insertion mutants. Bars represent means±s.d. (n=75, pooled from triplicate experiments). (f) Rescue of the leaf temperature decrease by the transformation of theblus1-1mutant withGFP-BLUS1. (g) Confocal images of GFP (green) and chlorophyll (red) fluorescence in guard cells of transgenic plants expressingGFP-BLUS1orGFPalone (upper panels). Lower panels show differential interference contrast images. The bars represent 5 μm. (h) Specific expression ofBLUS1in guard cell protoplasts (GC), as determined by RT–PCR analysis. MC, mesophyll cell protoplasts.KAT1andCBPwere used as guard cell and mesophyll cell markers, respectively.ACT8served as a control. Figure 2: Identification of the BLUS1 gene. ( a ) Map-based cloning of the BLUS1 gene. BLUS1 was mapped to the 290 kbp region between markers CER453585 and CER433575 on BAC clone FCAALL. Numbers indicate the recombination from a total of 170 chromosomes. ( b ) Genomic structure of the BLUS1 gene and sites of blus1 mutations. Black box indicates the protein-coding region. ( c ) Immunoblot analysis of BLUS1 protein in the blus1 mutants. The Rubisco large subunit (RbcL) was used as the loading control. Each lane contained 5 μg of guard cell proteins. ( d ) Impairment of the BL-dependent leaf temperature decrease of the blus1 T-DNA insertion mutants. The bar represents 1 cm. ( e ) Impairment of the BL-dependent stomatal opening in the epidermis of the T-DNA insertion mutants. Bars represent means±s.d. ( n =75, pooled from triplicate experiments). ( f ) Rescue of the leaf temperature decrease by the transformation of the blus1-1 mutant with GFP-BLUS1 . ( g ) Confocal images of GFP (green) and chlorophyll (red) fluorescence in guard cells of transgenic plants expressing GFP-BLUS1 or GFP alone (upper panels). Lower panels show differential interference contrast images. The bars represent 5 μm. ( h ) Specific expression of BLUS1 in guard cell protoplasts (GC), as determined by RT–PCR analysis. MC, mesophyll cell protoplasts. KAT1 and CBP were used as guard cell and mesophyll cell markers, respectively. ACT8 served as a control. Full size image BLUS1 phosphorylation is essential for stomatal opening BLUS1 showed an electrophoretic mobility shift induced by BL illumination; this response was absent in phot-deficient mutant ( Fig. 3a ), suggesting that BLUS1 might be phosphorylated by the phototropins. To address the phosphorylation status of BLUS1, we collected phosphopeptides from guard cell protoplasts by hydroxy acid-modified metal oxide chromatography [21] , [22] and analysed them by nanoLC-MS/MS. The amount of BLUS1 phosphopeptides increased after BL illumination ( Fig. 3b ). Moreover, the analysis indicated that the light-induced phosphorylation of BLUS1 occurred at the Ser-348 residue in the C-terminus ( Fig. 3c ). Consequently, we investigated the physiological role of Ser-348 phosphorylation in BLUS1. The WT BLUS1 gene complemented the blus1 phenotype, but mutation of Ser-348 to Ala (S348A) failed to complement the mutant phenotype ( Fig. 3e ). Furthermore, a kinase-dead mutant of BLUS1 in which Asp-157 was replaced with Asn (D157N) [23] did not rescue the blus1 phenotype ( Fig. 3e ). The production of the mutant proteins in the transgenic plants was independently verified ( Supplementary Fig. S3 ). We concluded that phosphorylation of Ser-348 as well as BLUS1 kinase activity is essential for BLUS1 signalling. As Ser-348 and the kinase domain are located in the C- and the N-terminus, respectively, the phosphorylation of Ser-348 may contribute to the regulation of kinase activity and/or to substrate recognition. Ser-348 is part of the consensus sequence motif, (RRISGWNF), which appears to be conserved in angiosperms, both monocots and dicots ( Supplementary Fig. S4 ). BLUS 1 appears to be a single gene in many plant species. We note that no protein kinases with this motif could be found in a representative bryophyte ( Physcomitella patens ) [24] or lycophyte ( Selaginella moellendorffii ) [25] . 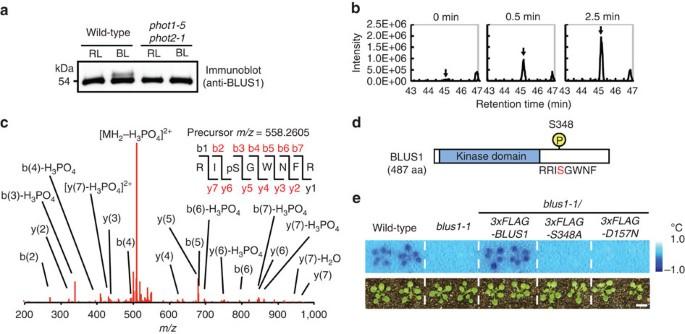Figure 3: The BL-dependent phosphorylation site in BLUS1. (a) BL-dependent electrophoretic mobility shift of BLUS1. The immunoblot was probed with anti-BLUS1 antibodies. Each lane contained 5 μg of guard cell proteins. (b,c) Phosphoproteome analyses of BL-dependent protein phosphorylation in guard cell protoplasts. Extracted ion chromatogram (b) and MS/MS spectrum (c) of the phosphopeptide corresponding to residues R346-R353 of BLUS1. (d) Schematic structure and phosphorylation site of BLUS1. RRISGWNF, a consensus motif around Ser-348. (e) Failure ofBLUS1 (S348A)andBLUS1 (D157N)to complement the defect in leaf temperature decrease in theblus1-1mutant. The bar represents 1 cm. Figure 3: The BL-dependent phosphorylation site in BLUS1. ( a ) BL-dependent electrophoretic mobility shift of BLUS1. The immunoblot was probed with anti-BLUS1 antibodies. Each lane contained 5 μg of guard cell proteins. ( b,c ) Phosphoproteome analyses of BL-dependent protein phosphorylation in guard cell protoplasts. Extracted ion chromatogram ( b ) and MS/MS spectrum ( c ) of the phosphopeptide corresponding to residues R346-R353 of BLUS1. ( d ) Schematic structure and phosphorylation site of BLUS1. RRISGWNF, a consensus motif around Ser-348. ( e ) Failure of BLUS1 (S348A) and BLUS1 (D157N) to complement the defect in leaf temperature decrease in the blus1-1 mutant. The bar represents 1 cm. Full size image Phototropins phosphorylate BLUS1 as a primary event We generated phosphospecific antibodies against pSer-348-BLUS1 (anti-pSer348) to examine BLUS1 phosphorylation more closely. BL-dependent phosphorylation of Ser-348 was found in the WT but not in the phot1 phot2 double mutant ( Fig. 4a ). Ser-348 phosphorylation was also detected in phot1 and phot2 single mutants ( Fig. 4a ), though the phot1 mutant displayed a lower degree of phosphorylation. Furthermore, blus1 phot1 and blus1 phot2 double mutants exhibited the same leaf temperature changes as the blus1 single mutant ( Fig. 4b ). Stomatal opening in these double mutants showed the impaired responses typical of the blus1 single mutant ( Fig. 4c ). These results indicated that signals from both phot1 and phot2 are transmitted to BLUS1. 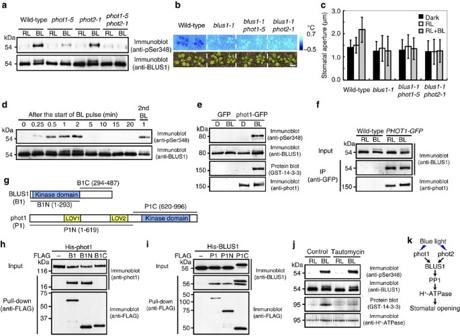Figure 4: Phosphorylation of BLUS1 by phototropins. (a) Phototropin-mediated phosphorylation of Ser-348 in BLUS1. The phosphorylation levels of Ser-348 were determined by immunoblotting using anti-pS348 antibodies. The amounts of BLUS1 proteins were determined using anti-BLUS1 antibodies. Each lane contained 5 μg of guard cell proteins. (b) Impairment of BL-dependent leaf temperature decrease in the double mutantsblus1 phot1andblus1 phot2. The bar represents 1 cm. (c) Impairment of BL-dependent stomatal opening in the double mutants. Bars represent means±s.d. (n=75, pooled from triplicate experiments). (d) Time course of BLUS1 phosphorylation levels on Ser-348 in response to BL. (e) Phosphorylation of BLUS1 on Ser-348 by phot1in vitro. GST-BLUS1 was expressed inE. coli. phot1-GFP was immunopurified from etiolated seedlings that had been illuminated with BL or kept in darkness (D). GST-BLUS1 was incubated with phot1-GFP in the presence of ATP, and BLUS1 phosphorylation was measured using anti-pS348 antibodies. Autophosphorylation of phot1 was detected by protein blotting using a 14-3-3 protein. Transgenic plants expressingGFPwere used as a control. (f) Co-immunoprecipitation of BLUS1 with phot1 in guard cells. Guard cell protoplasts (100 μg of proteins) expressingPHOT1-GFPwere illuminated with RL, and then a pulse of BL was applied. The proteins were immunoprecipitated with an anti-GFP antibody, and the immunoprecipitate was probed with anti-BLUS1 or anti-phot1 antibodies. Wild-type plants were used as controls. (g) Schematic structures of BLUS1 and phot1 used in pull-down assays. B1N; N-terminal fragment of BLUS1 (amino acids 1-294), B1C; C-terminal fragment of BLUS1 (294-487), P1N; N-terminal fragment of phot1 (1-619), P1C; C-terminal fragment of phot1 (620-996). (h,i) Pull-down assays of phot1 and BLUS1. All proteins were synthesized byin vitrotranscription/translation reactions. Indicated regions of FLAG-tagged BLUS1 were incubated with His-phot1 (h) and those of FLAG-tagged phot1 were incubated with His-BLUS1 (i). The proteins bound to anti-FLAG beads were detected using anti-phot1 (h), anti-BLUS1 (i) and anti-FLAG (h,i) antibodies. (j) Effect of 5 μM tautomycin on BL-dependent phosphorylation of BLUS1 and H+-ATPase. (k) Proposed pathway of BL signalling in guard cells. Figure 4: Phosphorylation of BLUS1 by phototropins. ( a ) Phototropin-mediated phosphorylation of Ser-348 in BLUS1. The phosphorylation levels of Ser-348 were determined by immunoblotting using anti-pS348 antibodies. The amounts of BLUS1 proteins were determined using anti-BLUS1 antibodies. Each lane contained 5 μg of guard cell proteins. ( b ) Impairment of BL-dependent leaf temperature decrease in the double mutants blus1 phot1 and blus1 phot2 . The bar represents 1 cm. ( c ) Impairment of BL-dependent stomatal opening in the double mutants. Bars represent means±s.d. ( n =75, pooled from triplicate experiments). ( d ) Time course of BLUS1 phosphorylation levels on Ser-348 in response to BL. ( e ) Phosphorylation of BLUS1 on Ser-348 by phot1 in vitro . GST-BLUS1 was expressed in E. coli . phot1-GFP was immunopurified from etiolated seedlings that had been illuminated with BL or kept in darkness (D). GST-BLUS1 was incubated with phot1-GFP in the presence of ATP, and BLUS1 phosphorylation was measured using anti-pS348 antibodies. Autophosphorylation of phot1 was detected by protein blotting using a 14-3-3 protein. Transgenic plants expressing GFP were used as a control. ( f ) Co-immunoprecipitation of BLUS1 with phot1 in guard cells. Guard cell protoplasts (100 μg of proteins) expressing PHOT1-GFP were illuminated with RL, and then a pulse of BL was applied. The proteins were immunoprecipitated with an anti-GFP antibody, and the immunoprecipitate was probed with anti-BLUS1 or anti-phot1 antibodies. Wild-type plants were used as controls. ( g ) Schematic structures of BLUS1 and phot1 used in pull-down assays. B1N; N-terminal fragment of BLUS1 (amino acids 1-294), B1C; C-terminal fragment of BLUS1 (294-487), P1N; N-terminal fragment of phot1 (1-619), P1C; C-terminal fragment of phot1 (620-996). ( h , i ) Pull-down assays of phot1 and BLUS1. All proteins were synthesized by in vitro transcription/translation reactions. Indicated regions of FLAG-tagged BLUS1 were incubated with His-phot1 ( h ) and those of FLAG-tagged phot1 were incubated with His-BLUS1 ( i ). The proteins bound to anti-FLAG beads were detected using anti-phot1 ( h ), anti-BLUS1 ( i ) and anti-FLAG ( h , i ) antibodies. ( j ) Effect of 5 μM tautomycin on BL-dependent phosphorylation of BLUS1 and H + -ATPase. ( k ) Proposed pathway of BL signalling in guard cells. Full size image We monitored the phosphorylation status of BLUS1 following a pulse of BL for 30 s at greater resolution. The phosphorylation of Ser-348 was initiated 15 s after the start of the pulse, reached a maximum within 1 min, and had returned to the initial dephosphorylated state by 5 min ( Fig. 4d ), with a re-phosphorylation of BLUS1 following a second pulse. The time course of BLUS1 phosphorylation revealed a more rapid response than described for H + -ATPase phosphorylation [12] , [26] and coincided with the timing of phot1 autophosphorylation [9] , [26] . Thus, it appeared conceivable that phototropins directly phosphorylate BLUS1. To test this possibility, we assayed BLUS1 phosphorylation in vitro by incubating recombinant BLUS1 with functional phot1-GFP with high purity from etiolated Arabidopsis seedlings that had been illuminated with BL ( Supplementary Fig. S5 ). In the presence of phot1-GFP, Ser-348 of BLUS1 became phosphorylated in a BL-dependent manner ( Fig. 4e ). Activation of phot1-GFP by BL was confirmed by 14-3-3 protein binding. Moreover, the BLUS1 protein co-immunoprecipitated with phot1-GFP from guard cells in the presence and absence of BL ( Fig. 4f ). Finally, we showed that phot1 directly interacted with BLUS1 in vitro by pull-down assays in which phot1 or BLUS1 proteins were used as bait ( Fig. 4h ). These findings confirmed that BLUS1 is an endogenous substrate of phototropin kinase. Next we investigated the site of interaction between phot1 and BLUS1 using N- and C-terminal fragments of these two recombinant proteins ( Fig. 4g ). Full-length phot1 interacted with the BLUS1 N-terminus, which includes the kinase domain ( Fig. 4h ). Full-length BLUS1 interacted with both the N- and C-termini of phot1, including the photosensory LOV and kinase domains, respectively ( Fig. 4i ). Interestingly, immunoblot analysis indicated that the phot1 kinase lacking the LOV domains (P1C) induced a mobility shift of BLUS1 ( Fig. 4i ) due to the phosphorylation of Ser-348 in the dark ( Supplementary Fig. S6 ). In contrast, the full-length phot1 affected BLUS1 mobility only slightly ( Fig. 4i ). We concluded that the C-terminus containing the phot1 kinase phosphorylates BLUS1 at the physiological site, and that the LOV domains act as inhibitors of the kinase activity, as has been reported from a model system in which the LOV2 domain inhibits in vitro casein phophorylation by phot2 kinase [27] . As BLUS1 is a Ser/Thr protein kinase, it could be hypothesized to directly phosphorylate the H + -ATPase in guard cells. However, Fc induced H + -ATPase phosphorylation in blus1 mutants as well as WT plants ( Fig. 1h ), suggesting an involvement of protein kinases other than BLUS1. To identify the role of BLUS1 in this pathway, we tested the effects of tautomycin, an inhibitor of PP1, on the BL-dependent phosphorylation of BLUS1 and H + -ATPase. The inhibitor suppressed H + -ATPase phosphorylation, but had no effects on BLUS1 phosphorylation ( Fig. 4j ). BLUS1 therefore appears to precede PP1 in the signalling pathway for stomatal opening ( Fig. 4k ). blus1 mutants decrease stomatal conductance and CO 2 fixation As blus1 mutants are defective solely in BL-dependent stomatal opening ( Fig. 1 and Supplementary Fig. S2 ), they offer an excellent system to assess how the stomatal BL response contributes to photosynthetic CO 2 assimilation under natural light conditions. We compared the stomatal conductance and photosynthetic CO 2 assimilation between WT and blus1 under white light at 1,000 μmol m −2 s −1 and well-watered conditions. As expected, stomatal conductance was strongly reduced in blus1 compared with the WT at 350 p.p.m. CO 2 ( Fig. 5a ), but their rates of photosynthetic CO 2 assimilation were indistinguishable ( Fig. 5b ). Upon transfer to darkness, blus1 mutants showed a slower decrease in conductance than WT plants and did not close stomata completely within 30 min ( Fig. 5a ). The conductance was enhanced significantly in the WT but only slightly increased in blus1 when the CO 2 concentration was reduced to 200 p.p.m. ( Fig. 5c ); the net assimilation rate was two-fold higher in WT than in blus1 ( Fig. 5d ). The greater enhancement of stomatal aperture in response to decreased CO 2 in the WT compared with blus1 is partly due to that the BL-specific response of stomata is stimulated by low intercellular concentration of CO 2 (ref. 28 ). 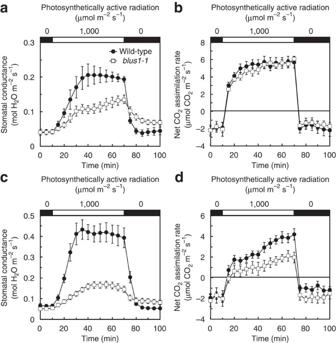Figure 5:blus1mutants decrease stomatal conductance and CO2fixation (a,c) Stomatal conductance in response to white light (1,000 μmol m−2s−1). The bars represent means±s.e.m. (n=5). (b,d) Photosynthetic CO2assimilation rate in response to white light. (a,b) 350 p.p.m. CO2. (c,d) 200 p.p.m. CO2. The bars represent means±s.e.m. (n=5). Figure 5: blus1 mutants decrease stomatal conductance and CO 2 fixation ( a , c ) Stomatal conductance in response to white light (1,000 μmol m −2 s −1 ). The bars represent means±s.e.m. ( n =5). ( b , d ) Photosynthetic CO 2 assimilation rate in response to white light. ( a , b ) 350 p.p.m. CO 2 . ( c , d ) 200 p.p.m. CO 2 . The bars represent means±s.e.m. ( n =5). Full size image We demonstrated that the phosphorylation of Ser-348 in BLUS1 was essential for the activation of the H + -ATPase to drive stomatal opening, and concluded that BLUS1 was a substrate for phototropin kinase and that its phosphorylation was a primary event in phototropin signalling. Two potential substrates for phototropin kinase that are involved in phototropism have been identified, namely the auxin efflux transporter ATP-binding cassette B19 (ref. 29 ) and phytochrome kinase substrate 4 (ref. 30 ). However, neither the site of phosphorylation nor the nature of the role in phototropism is known for these two proteins. To our knowledge, BLUS1 is the first identified phototropin substrate with a known essential role in phototropin-mediated signalling. Phototropins mediate a wide range of plant responses, including phototropism, chloroplast relocation, leaf flattening, leaf positioning and stomatal opening. It still remains an open question as to how phototropins bring about a diverse set of BL responses in plants [7] , [8] , [10] . We demonstrated that mutation of the BLUS1 gene does not affect any of the other phototropin-mediated responses tested ( Supplementary Fig. S2 ). Furthermore, no common components except phototropins have been found in the signalling pathways of phototropism, chloroplast movements and stomatal opening [8] . Apparently, several BL signalling pathways diverge from a component just downstream of the phototropins. The blus1 mutant exhibits loss of stomatal BL response ( Fig. 1 ) and shows slow and incomplete stomatal closure when the plants are transferred to darkness ( Fig. 5a ). These properties of blus1 mutants resemble those of ferns that lack stomatal BL responses and exhibit slow and incomplete stomatal closure upon darkness [2] , [31] . As a large decrease in the atmospheric CO 2 concentration occurred during the Devonian and Carboniferous periods, the time when seed plants evolved [32] , the acquisition of stomatal BL responses may have conferred competitive advantages over plants lacking these responses. Plant materials and growth conditions The Arabidopsis thaliana ecotype Columbia was used in all experiments. Ethyl methanesulfonate-mutagenized M2 seeds were purchased from Lehle Seeds or prepared by the Nisshoku Group. The phot1-5 , phot2-1 and phot1-5 phot2-1 mutants and transgenic PHOT1-GFP plants have been described elsewhere [33] , [34] , [35] . blus1-3 (SALK_000221) and blus1-4 (GABI_222H02) were obtained from the Nottingham Arabidopsis Stock Center (NASC), Nottingham, UK and GABI-Kat, respectively. For the mutant screen, plants were grown for 11 days on 0.8% (w/v) agar plates containing half-strength Murashige–Skoog salts (pH 5.7), 2.3 mM MES and 1% (w/v) sucrose under continuous white light (60 μmol m −2 s −1 ) at 23 °C. The plants were then transferred to a soil:vermiculite (1:1) mixture and further grown under a 13/11 h light/dark cycle for 9 days. For some experiments, the plants were grown on soil:vermiculite (1:1) for 4 weeks under a 14/10 h light/dark cycle. Mutant screen by thermal imaging Leaf temperature was determined by infrared thermography (TVS-8500, NEC Avio Infrared Technologies). Plants were kept in the dark overnight at 21–24 °C with 40–50% relative humidity and were then illuminated with RL (80 μmol m −2 s −1 ) for 50 min. Then, a weak continuous BL (5 μmol m −2 s −1 ) was superimposed on the RL. The RL was obtained by passing light from a red fluorescent lamp (FL40S R, Panasonic) through a colour filter (no. 22, Tokyo Butai Showmei), and the BL was provided by a light-emitting diode (5050ML60-W/B). Temperature decreases were visualized using thermal images, which were obtained by the subtraction of an image taken before the start of BL irradiation from one taken after 15 min of BL irradiation using PE Professional software (NEC Avio Infrared Technologies). Stomatal aperture and gas exchange The stomatal aperture in the abaxial epidermis was measured by microscopic examination (Eclipse TS100; Nikon) [11] . Stomatal conductance and photosynthetic CO 2 assimilation were determined using a gas-exchange system (LI-6400, Li-Cor) [18] . Isolation of guard cell protoplasts Guard cell protoplasts were prepared enzymatically from leaves [19] , [36] . A typical yield of guard cell protoplasts was 4.3 × 10 7 cells (1,000 μg proteins) per 5,000 leaves [19] . Measurement of H + pumping BL- and Fc-dependent H + pumping were determined with a glass pH electrode as described previously [19] . The reaction mixture (0.8 ml) contained 0.125 mM MES-NaOH (pH 6.0), 1 mM CaCl 2 , 0.4 M mannitol, 10 mM KCl and guard cell protoplasts (50–80 μg proteins). Immunoblot and protein blot analyses Guard cell protoplasts were illuminated with RL (600 μmol m −2 s −1 ) for 30 min, and then a pulse of BL (100 μmol m −2 s −1 , 30 s) was superimposed. To detect phototropins and BLUS1, the phosphorylation reaction was terminated at 2 min after the start of the BL pulse by adding trichloroacetic acid (TCA) to the guard cell protoplast suspension. For the H + -ATPase, the phosphorylation was terminated at 3.5 min after the pulse as described previously [12] . Immunoblotting was performed according to Kinoshita and Shimazaki [12] , with slight modifications. We generated antibodies against the C-terminal region and phosphorylated Ser-348 of BLUS1 by immunizing rabbits with recombinant GST-BLUS1 (K294-G487) and a synthetic phospho-BLUS1 peptide (KNRRIpSGWNF), respectively. Antibodies against phot1, phot2 and H + -ATPase were described previously [12] , [18] , [19] . Phosphorylation levels of phot1 and the H + -ATPase were determined by protein blotting using GST-14-3-3 (refs 12 , 36 ). Phosphoproteome analysis TCA-treated guard cell proteins (100 μg) were suspended in 0.1 M Tris-HCl (pH 8.0) containing 8 M urea, protein phosphatase inhibitors and a protease inhibitor cocktail (Sigma-aldrich), and the suspension was sonicated for 5 min. The proteins were reduced by dithiothreitol, alkylated with iodoacetamide and digested with Lys-C, followed by trypsin treatment [37] . The digested samples were desalted using stage tips with C18 Empore disk membranes (3M) [38] . The samples were enriched for phosphopeptides by hydroxy acid-modified metal oxide chromatography using lactic acid-modified titania [21] , [22] . Briefly, the digested samples were diluted with 0.1% TFA, 80% acetonitrile containing 300 mg ml −1 lactic acid (solution A), and then loaded to custom-made metal oxide chromatography tips preliminary equilibrated with solution A. After successive washing with solution A, and then 0.1% TFA and 80% acetonitrile, the peptides were eluted with 0.5% piperidine. The phosphopeptide fractions were desalted and concentrated using a vacuum evaporator and then subjected to nanoLC-MS/MS analyses using LTQ-Orbitrap (Thermo Fisher Scientific) [39] . Peptides and proteins were identified by automated database searches using Mascot version 2.3 (Matrix Science) in the TAIR database (release 10), with a precursor mass tolerance of 3 p.p.m., a fragment ion mass tolerance of 0.8 Da, and strict trypsin specificity allowing for up to two missed cleavages. Cysteine carbamidomethylation was set as a fixed modification. Methionine oxidation serine, threonine and tyrosine phosphorylations were allowed as modifications. Generation of transgenic plants The 3,965 bp genomic sequence, including the promoter, coding region and 3′-UTR region of BLUS1 , was amplified using primers 5′-CGGTATCGATAAGCTTGCTTTAGGAATGTTGAAAGTATTCAGAG-3′ and 5′-TAGAACTAGTGGATCCTCGCCTGTAGTCACTTGGCAC-3′. The product was subcloned into the pBluescript II KS (+) (Stratagene) using the In-Fusion system (Clontech). The GFP or 3xFLAG sequence was inserted after the start codon of BLUS1 , and the resulting GFP-BLUS1 or 3xFLAG-BLUS1 fragment was introduced into the Hind III/ Bam HI site of the pRI 101-AN (Takara). Each construct was transformed into blus1-1 plants using Agrobacterium tumefaciens . Point mutations Site-directed mutagenesis was performed using the QuikChange Site-Directed Mutagenesis Kit (Stratagene). The primers used were 5′-TAGTGAAGAATAGAAGAATCGCTGGGTGGAATTTCCGTGAAG-3′ and 5′-CTTCACGGAAATTCCACCCAGCGATTCTTCTATTCTTCACTA-3′ for BLUS1-S348A , and 5′-GATCCGTGAAGCTCGCTAATTTCGGAGTATCTGCA-3′ and 5′-TGCAGATACTCCGAAATTAGCGAGCTTCACGGATC-3′ for BLUS1-D157N . Localization of GFP-BLUS1 Fluorescent images were obtained using a confocal laser-scanning microscope (Digital Eclipse C1; Nikon) [14] . The wavelengths of excitation and emission for GFP were 488 nm and 515–530 nm, and those for chlorophyll fluorescence were 543 and 590 nm long-pass. RT–PCR analysis Total RNA was extracted from guard cell and mesophyll cell protoplasts using ISOGEN (Nippon Gene) and RNeasy (Qiagen). First-strand cDNA was synthesized from 1 μg of total RNA using the SuperScript III First-strand Synthesis System (Invitrogen). The primer sets used for PCR were 5′-ATGGCTCGGAACAAGCTCGAG-3′ and 5′-TTAACCCAAAACACTATCTTTATCAGCAC-3′ for BLUS1 ; 5′-ACTTTACGCCAGTGGTCGTACAAC-3′ and 5′-AAGGACTTCTGGGCACCTGAATCT-3′ for ACT8 ; 5′-ATGTCGATCTCTTGGACTCG-3′ and 5′-CTTGAAGCAAACTCTGAAGCAGCTC-3′ for KAT1 ; 5′-ATGGGTCTTGAAGTTGGGTCCTTATG-3′ and 5′-TGCAGAACACTTCTAGGGTGTTTCTC-3′ for CBP1 . In vitro phosphorylation assay Full-length BLUS1 was subcloned into the pGEX-2T (GE Healthcare) and introduced into E. coli strain Rosetta-gami B (Merck). The GST-BLUS1 was purified using glutathione–Sepharose (GE Healthcare). phot1-GFP was obtained by immunoprecipitation from of 3-day-old etiolated seedlings that had been illuminated with BL (100 μmol m −2 s −1 ) for 1 min or kept in darkness. 1,500 etiolated seedlings were ground in extraction buffer containing 50 mM MOPS-KOH (pH 7.5), 2.5 mM EDTA, 100 mM NaCl, 0.5 mM PMSF, 10 μM leupeptin, 2 mM DTT, 10 mM NaF, 0.5 mM ammonium molybdate and 100 nM calyculin A. Following centrifugation at 10,000 g for 10 min, the resulting supernatant was centrifuged at 100,000 g for 1 h and microsomal membranes were obtained as a pellet. The membranes (250 μg proteins) were resuspended in extraction buffer with 0.1% Triton X-100, and kept on ice for 10 min. After centrifugation at 10,000 g for 10 min, the supernatant was used for immunoprecipitation using the GFP-Trap (Chromotek). After incubation for 1 h, the beads were washed three times and immunopurified phot1-GFP was used for phosphorylation assay. The phosphorylation of GST-BLUS1 by phot1-GFP on beads was performed in a reaction mixture containing 25 mM Tris-HCl (pH 7.4), 10 mM MgCl 2 and 100 μM ATP at 30 °C for 2 h under BL (100 μmol m −2 s −1 ) or in darkness. The phosphorylated GST-BLUS1 proteins were subjected to immunoblotting using anti-pSer348 and anti-BLUS1 antibodies. Co-immunoprecipitation assay Guard cell protoplasts (100 μg proteins) were mixed with an equal volume of medium containing 100 mM MOPS-KOH (pH 7.5), 5 mM EDTA, 200 mM NaCl, 1 mM PMSF, 20 μM leupeptin, 4 mM DTT, 20 mM NaF, 1 mM ammonium molybdate, 200 nM calyculin A and 0.4% Triton X-100, and kept on ice for 10 min. Following centrifugation at 10,000 g for 10 min, the supernatant was reacted with GFP-Trap for 1 h. After washing the GFP-Trap three times, immunoprecipitated proteins were detected using anti-BLUS1 and anti-phot1 antibodies. In vitro pull-down assay His-tagged and FLAG-tagged proteins were synthesized using an in vitro transcription/translation system (BioSieg). The protein pair used for the assay was produced in a single tube. Fifty microliter of the synthesized proteins were mixed with 450 μl binding buffer containing 20 mM Tris-HCl (pH 7.4), 140 mM NaCl and 0.1% Triton X-100, and were kept on ice for 10 min. After centrifugation at 10,000 g for 10 min, the supernatants were mixed with anti-FLAG M2 agarose (Sigma-Aldrich), and incubated for 1 h. After washing the beads three times, the bound proteins were subjected to immunoblotting using anti-phot1 and anti-BLUS1 antibodies. FLAG-tagged proteins were detected using anti-FLAG (Sigma-Aldrich) and TrueBlot secondary antibodies (Rockland Immunochemicals). Phylogenetic analysis All sequence data were obtained from the phytozome homepage ( http://www.phytozome.net ). Sequence alignment was performed using the ClustalW program with default parameters (gap opening penalty, 10; gap extension penalty, 0.2; delay divergent cutoff, 30%). Phylogenetic analysis was done using the MEGA software, version 5, with the neighbour-joining method [40] . All positions containing gaps and missing data were eliminated from the data set. The number of bootstrap replicates was 1,000. How to cite this article: Takemiya A. et al. Phosphorylation of BLUS1 kinase by phototropins is a primary step in stomatal opening. Nat. Commun. 4:2094 doi: 10.1038/ncomms3094 (2013).